Analysis ofopo cis-regulatory landscape uncovers Vsx2 requirement in early eye morphogenesis The self-organized morphogenesis of the vertebrate optic cup entails coupling the activation of the retinal gene regulatory network to the constriction-driven infolding of the retinal epithelium. Yet the genetic mechanisms underlying this coordination remain largely unexplored. Through phylogenetic footprinting and transgenesis in zebrafish, here we examine the cis -regulatory landscape of opo , an endocytosis regulator essential for eye morphogenesis. Among the different conserved enhancers identified, we isolate a single retina-specific element (H6_10137) and show that its activity depends on binding sites for the retinal determinant Vsx2. Gain- and loss-of-function experiments and ChIP analyses reveal that Vsx2 regulates opo expression through direct binding to this retinal enhancer. Furthermore, we show that vsx2 knockdown impairs the primary optic cup folding. These data support a model by which vsx2 , operating through the effector gene opo , acts as a central transcriptional node that coordinates neural retina patterning and optic cup invagination in zebrafish. The organogenesis of the vertebrate eye is a complex process that involves the precise integration of inductive signals, intrinsic genetic programs and morphogenetic movements. As the general vertebrate body plan is established, the main architecture of the eye is acquired in the developmental window comprised between the specification of the eye field at early gastrulation and the onset of neuronal differentiation at pharyngula stage [1] , [2] . During this period, an initially undifferentiated mass of precursor cells in the anterior neural plate differentiates into the neural retina, the retinal pigmented epithelium (RPE) and the optic stalk domains. Signalling molecules emanating from adjacent tissues (for example, SHH from the midline, activins from the extraocular mesenchyme and fibroblast growth factors (FGFs) from the presumptive lens) activate domain-specific transcriptional regulators, which in turn restrict the precursors’ potentiality and specify the features of the different eye subdivisions [2] , [3] , [4] . The formation of defined boundaries between adjacent domains often depends on reciprocal transcriptional repression. This mechanism is exemplified by the mutual repression between Pax2/Pax6, which helps defining the border between optic stalk and optic cup [5] . The neural retina domain is specified in the distal optic vesicle under the influence of FGFs, derived either from the lens ectoderm or the neuroepithelium itself [6] , [7] , [8] , [9] . In a number of vertebrate models, ectopic activation of the FGF–MAPK pathway seems to be sufficient to transdifferentiate the RPE into retina. This transformation involves the general downregulation of the RPE gene regulatory network, particularly the repression of a key specifier, the bHLH TF Mitf [3] , [10] , [11] . The gene encoding for the homeodomain TF Vsx2, formerly known as Chx10 , is the earliest domain-specific marker expressed in the presumptive neural retina [12] . Initial analysis of Vsx2 function described that its mutation in mice ( ocular retardation , or j ) resulted in microphthalmia, and revealed its essential role in neuroepithelial proliferation and bipolar cells differentiation [13] . Similar phenotypes were also observed in human Vsx2 mutations [14] and in vsx2 -depleted embryos in zebrafish [15] , [16] . More recent studies on early stages of eye development have shown that Vsx2 represses Mitf and hence RPE identity, thus acting as a central component of the gene regulatory network involved in the specification of the neural retina domain [17] , [18] , [19] , [20] . Interestingly, the FGF-induced reprogramming of the RPE lineage does not occur in null mutant mice for Vsx2 (ref. 18 ), thus indicating that Vsx2 is an essential downstream node in the MAPK–FGF pathway, responsible for neural retina determination. As tissue patterning takes place, eye precursors within their different domains undergo a coordinated series of morphogenetic movements that shape the primordium into a hemispheric optic chamber [21] , [22] , [23] . Two major characteristic movements have been described by anatomical observations and live-imaging recordings in all vertebrate models. The first, known as evagination, results in the formation of bilateral optic vesicles either by the lateral bulging of coherent epithelial sheets, as reported in tetrapods [24] , [25] , or by the rearrangement of individual cells, as described in teleost models [26] , [27] . In a second series of coordinated movements (that is, invagination), the neural retina and RPE domains fold to form a bilayered cup that covers the lens vesicle, which simultaneously invaginates from the surface ectoderm [21] , [25] , [28] . Although contractile interepithelial filopodia have been shown to participate in the fine-tuning mechanism that coordinates optic cup and lens morphogenesis [29] , a number of studies indicate that both tissues fold following cell intrinsic-independent mechanisms. Recent data in mice have shown that the invagination of the lens ectoderm is achieved through an apical constriction mechanism driven by the RhoA-dependent activation of the actin regulator Shroom3 (refs 30 , 31 ). In contrast, the inward folding of the neural ectoderm has been described, both in mammals and teleosts, as a tissue-autonomous mechanism depending on integrin function [28] , [32] . Mutant analysis in medaka ( Oryzias latipes ) has identified the vertebrate-specific transmembrane protein Opo, encoded by the gene ojoplano ( opo ), as an essential component of the molecular machinery involved in neural retina morphogenesis [28] , [33] . Opo is a hypomorphic splicing mutation that results in a premature stop codon in a fraction of the mature transcripts, and thus in a reduction of wild-type protein levels. In opo mutants, focal adhesion components are not efficiently recruited to the basal surface of the retinal neuroepithelium and the folding of the optic cup is severely impaired [28] . More recently, biochemical analyses have shown that Opo controls the polarized endocytosis of integrins through interference with the clathrin adaptors Numb and Numbl (ref. 34 ). It seems a logical assumption that tissue patterning and morphogenetic movements are coordinated phenomena. Yet little is known about the molecular link between transcriptional specifiers and morphogenetic effectors during eye development [35] , [36] . Here we perform a comprehensive analysis of the genomic landscape of the morphogenetic regulator opo. Through a combination of phylogenetic footprinting, analysis of epigenetic marks and transgenesis assays in zebrafish, we explore the regulatory input onto the opo promoter. Among the nine tissue-specific enhancers identified, H6_10137 exclusively drives the expression in the neural retina domain. We show that regulatory activity by H6_10137 depends on evolutionarily conserved Vsx2-binding sites, and demonstrate the physical interaction between Vsx2 and the eye enhancer in vivo . Furthermore, we show that vsx2 regulates opo expression both in gain- and loss-of-function experiments. Finally, vsx2 morpholino knockdown in zebrafish results in a range of eye malformations, including microphthalmia and optic cup folding defects resembling the ocular phenotype of opo mutants. In addition to its well-established role as a specifier of the retinal domain, our data indicate a role for Vsx2 in optic cup morphogenesis. According to our model, vsx2 would act as a genetic hub that coordinates neural retina patterning and morphogenesis in the developing zebrafish eye. Identification of CNEs in the opo locus The developmental gene opo plays an essential role during the morphogenesis of a number of tissues including the eye, brain, heart, fins and neural crest derivatives [28] . Opo is present as a single copy in the genome of all vertebrates studied and, together with its neighbor genes tfap2a and slc35b3 , forms a relatively large syntenic block ( ∼ 2 Mb in mammalian genomes). Its human orthologue, also known as orofacial cleft candidate 1 ( ofcc1 ) is located at the distal region of chromosome 6p (6p23.4). This region has been associated to hereditary congenital diseases such as orofacial clefting [37] , schizophrenia [38] and Tourette syndrome [39] . To gain insight into the opo regulatory logic, we first used a phylogenetic footprinting approach to detect potential cis -regulatory elements conserved among vertebrate genomes. Using Vista alignment tools, we identified and cloned a collection of 23 highly conserved (≥70% identity from mammals to teleosts) non-coding elements (CNEs) distributed throughout the human locus ( Fig. 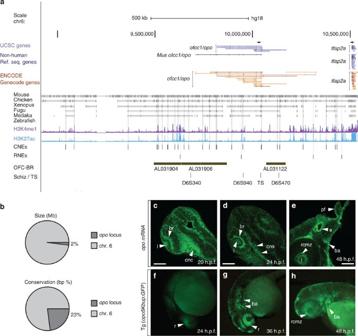Figure 1:Opolandscape. (a) Representation of theopolandscape in 6p24.3 of the human genome (NCBI36/hg18), showingopo/orofacial clefting candidate 1(opo/ofcc1) and TFap-2 alpha(tfap2a). The sequence conservation among six vertebrate species (grey) is represented above. The sum of H3K4me1 and H3K27ac marks for human cell lines are shown in light blue and purple, respectively. Both conserved CNEs and non-conserved reference elements (RNEs) are indicated in dark blue bars. The CNE marked in grey was not screened for enhancer activity. Orofacial clefting break-point regions (OFC), Tourett syndrome mutation (TS: chr6:10041064) and Schizophrenia-linked (Schiz) markers are also represented. (b) Theopolocus represents 2% of the size (Mb) of the chromosome six and contains 23% of all the non-coding highly conserved elements in this chromosome. Non-coding highly conserved bp in the locus versus non-coding highly conserved bp in the rest of the chromosome are represented. (c–e) Whole-mount FISH show the localization ofopotranscripts in basal retina (br), cranial neural crest (cnc), ear (e), lens (l), central nervous system (cns), retina ciliar marginal zone (rcmz), pharyngeal arches (pa) and in the epidermal ridge of the pectoral fins (pf). (f–h) GFP expression of the stable transgenic lineTg(opo5kbup:GFP) in retina (r), cranial neural crest (cnc), pharyngeal arches (ba) and retina ciliary marginal zone (rcmz). 1a ; Supplementary Table 1 ). Interestingly, although the genomic region including opo covers only 2% of the chromosome 6, it contains 23% of the CNEs within this chromosome ( Fig. 1b ). This suggests that opo has a complex regulatory input, as previously reported for other developmental genes [40] . For each CNE, we then examined the co-occurrence of the predictive enhancer epigenetic marks H3K4me1 and H3K27ac, as determined in previous chromatin immunoprecipitation (ChIP)-Seq studies in human cell lines [41] , [42] and, for their homologous regions, in zebrafish embryos [43] . 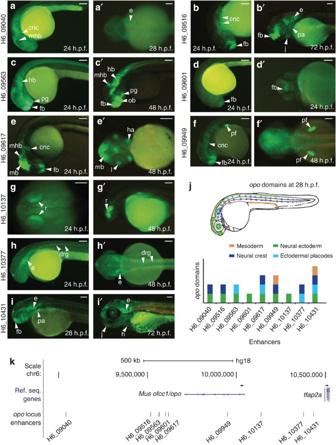Figure 2:Opolocus enhancers. (a–i) GFP expression is shown at early (24–28 h.p.f.) and late (48–72 h.p.f.) developmental stages for each of the enhancers identified in theopolocus. The offspring of one representative founder (F1) is shown for each enhancer (see also,Table 1andSupplementary Table 3for a full description). Arrowheads: midbrain–hindbrain boundary (mhb); pharyngeal arches (pa); forebrain (fb); ear (e); jaw (j); hindbrain (hb); midbrain (mb); pituitary gland (pg); olfactory bulbs (ob); hyoid arch (ha); lens (l); pectoral fin (pf); retina (r); dorsal root ganglia (drg); heart (h). (j) The zebrafish model is coloured according to the sum of the enhancers’ GFP patterns. The total sum of theopolocus enhancers’ patterns recapitulates most of theopoexpression domains at 28 h.p.f. (k) Relative localization on the enhancers inopolocus. Scale bar, 100 μm. These analyses revealed that a large majority of the identified CNEs (21 out of 23) overlap with regions labelled with at least one epigenetic mark, either in human cell lines, zebrafish embryos or both ( Supplementary Table 2 ), suggesting that these conserved regions may act as enhancers. As a reference, four non-conserved elements (named here H6_09628, H6_09941, H6_10309 and H6_10455) tagged with H3K4me1 and H3K27ac marks in human cell lines ( Fig. 1a ) were also cloned and included in further analyses. Figure 1: Opo landscape. ( a ) Representation of the opo landscape in 6p24.3 of the human genome (NCBI36/hg18), showing opo/orofacial clefting candidate 1 ( opo/ofcc1 ) and TF ap-2 alpha ( tfap2a ). The sequence conservation among six vertebrate species (grey) is represented above. The sum of H3K4me1 and H3K27ac marks for human cell lines are shown in light blue and purple, respectively. Both conserved CNEs and non-conserved reference elements (RNEs) are indicated in dark blue bars. The CNE marked in grey was not screened for enhancer activity. Orofacial clefting break-point regions (OFC), Tourett syndrome mutation (TS: chr6:10041064) and Schizophrenia-linked (Schiz) markers are also represented. ( b ) The opo locus represents 2% of the size (Mb) of the chromosome six and contains 23% of all the non-coding highly conserved elements in this chromosome. Non-coding highly conserved bp in the locus versus non-coding highly conserved bp in the rest of the chromosome are represented. ( c – e ) Whole-mount FISH show the localization of opo transcripts in basal retina (br), cranial neural crest (cnc), ear (e), lens (l), central nervous system (cns), retina ciliar marginal zone (rcmz), pharyngeal arches (pa) and in the epidermal ridge of the pectoral fins (pf). ( f – h ) GFP expression of the stable transgenic line Tg(opo5kbup:GFP ) in retina (r), cranial neural crest (cnc), pharyngeal arches (ba) and retina ciliary marginal zone (rcmz). Full size image The distribution of opo transcripts during development has been described both in mouse and medaka tissues [28] , [33] , but not in zebrafish, the model system used for functional analyses in this study. To extend our observations to zebrafish embryos, we performed fluorescent in situ hybridization analyses at stages 20, 24 and 48 h.p.f. ( Fig. 1c–e ). In agreement with previous data in other vertebrates, opo mRNA localized mainly at the basal side of the retinal epithelium, lens, brain and neural crest precursors at early stages (20–24 h.p.f. ; Fig. 1c,d ; Supplementary Fig. 1 ). Later on, at 48 h.p.f., opo expression appeared more prominent at the retinal ciliary marginal zone, pharyngeal arches, inner ear and pectoral fins ( Fig. 1e ; Supplementary Fig. 1 ). Using these observations as a reference, we then examined whether the genomic region found immediately upstream of the opo transcription start site contained enough regulatory information to recapitulate the entire expression pattern of the gene. To answer this question, we took advantage of the compact genome size in medaka (800 Mb), as well as the precise annotation of the opo transcription start site in this species. A 5.6-kb fragment, containing both the medaka promoter of the gene and some proximal elements (that is, including the homologous regions of the human CNEs here termed H6_10126 and H6_10137), was cloned into a reporter (enhanced green fluorescent protein (eGFP)) vector and screened in transgenic assays in zebrafish. The examination of the stable lines ( n =3) generated by the injection of the Tg(opo5Kbup:GFP) construct showed that the opo proximal region drives the reporter expression to the developing eye and pharyngeal arches ( Fig. 1f–h ). Although these tissues comprise a significant part of the whole opo expression pattern, the proximal 5.6-kb element failed to drive the reporter into several domains (for example, the early migratory cephalic neural crest, lens, brain and pectoral fins). This observation suggests that additional cis -regulatory elements cooperate to control opo transcription. Functional identification of opo enhancers To investigate whether some of the identified CNEs behave as active enhancers, we tested them individually by transgenesis analysis in zebrafish. In these experiments, we used the zebrafish enhancer detector system (ZED), a Tol2-mediated transgenesis shuttle that includes a minimal promoter linked to GFP and a cardiac-actin:RFP (red fluorescent protein) cassette as an internal control for transgenesis [44] . The progeny (F1) of the putative transgenic fish (founders) was screened for the reporter expression between 24 and 72 h.p.f. 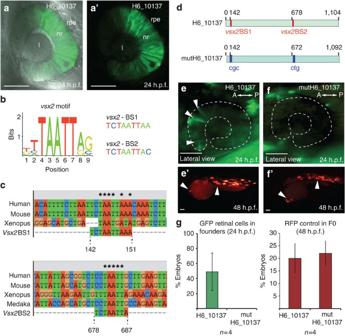Figure 3: Identification of Vsx2-binding sites in H6_10137. (a,a′) Confocal section shows GFP expression driven by the H6_10137 enhancer in the neural retina. (l) lens, (nr) neural retina and (rpe) RPE. (b) Positional weight matrix showing Vsx2-binding motif. Both Vsx2 DNA-binding sites (BS1 and BS2) located within the H6_10137 sequence are represented. (c) Multispecies alignment of H6_10137 enhancer showing sequence conservation of BS1 and BS2 (Human—NCBI36/hg18; Mouse—NCBI37/mm9; Xenopus—JGl 4.2/xenTro3; Medaka—MEDAKA1/oryLat2). (d) Both Vsx2 DNA-binding sites were mutated generating the construct mutH6_10137 (e) H6_10137 mosaic transgenic embryo (F0) expressing GFP in retina neuroblasts (arrowheads). (f) mutH6_10137 transgenic embryo (F0) showing no GFP activity in the retina. (e′,f′) RFP trangenesis controls were observed for both constructs in the heart and somites at 48 h.p.f. (arrowheads). (g) Percentages of GFP retina cells for both H6_10137 and mutH6_10137 constructs and its respective controls. Four independent experiments were carried out for a total number of scored embryos injected with the control (H6_10137,n=580) or the mutated (mutH6_10137,n=580) constructs. Error bars indicate s.d. of the mean. Scale bar, 50 μm in (a,a′,e,f) and 100 μm in (e′,f′). ( Supplementary Table 3 ). We observed that 12 out of the 23 CNEs tested (52%) were able to activate the GFP expression. In contrast, none of the four non-conserved elements marked for H3K4me1 and H3K27ac behaved as an enhancer in the developmental window considered in our screen. Among the 12 positives CNEs, we found an irreproducible GFP pattern between founders in three cases, suggesting that these elements either do not act as specific enhancers or require additional regulatory information to be active. The remaining nine consistently directed distinct tissue-specific expression patterns in several independent founders (three or more), and were considered functional enhancers ( Supplementary Table 3 ). Several of these elements directed reporter expression in the brain or craniofacial derivatives ( Fig. 2a–i ), whereas other territories such as the lens or the fins were the targets of a single enhancer ( Fig. 2e,f ). Significantly, we identified only a single enhancer, H6_10137, driving the reporter expression in the neural retina domain ( Fig. 2g ). A detailed description of the expression domains controlled by each individual enhancer is shown in Table 1 and summarized in Fig. 2j . Most of the enhancers were located either 5′ or 3′ of the opo transcriptional unit, and a single intronic enhancer, H6_09949, was identified ( Fig. 2k ). Interestingly, four of the identified elements, H6_09516, H6_09601, H6_09949 and H6_10137, belong to the collection of 557 ancient pan-vertebrate aCNEs conserved both in cartilaginous and bony vertebrate lineages [45] . Figure 2: Opo locus enhancers. ( a – i ) GFP expression is shown at early (24–28 h.p.f.) and late (48–72 h.p.f.) developmental stages for each of the enhancers identified in the opo locus. The offspring of one representative founder (F1) is shown for each enhancer (see also, Table 1 and Supplementary Table 3 for a full description). Arrowheads: midbrain–hindbrain boundary (mhb); pharyngeal arches (pa); forebrain (fb); ear (e); jaw (j); hindbrain (hb); midbrain (mb); pituitary gland (pg); olfactory bulbs (ob); hyoid arch (ha); lens (l); pectoral fin (pf); retina (r); dorsal root ganglia (drg); heart (h). ( j ) The zebrafish model is coloured according to the sum of the enhancers’ GFP patterns. The total sum of the opo locus enhancers’ patterns recapitulates most of the opo expression domains at 28 h.p.f. ( k ) Relative localization on the enhancers in opo locus. Scale bar, 100 μm. Full size image Table 1 Expression domains of the enhancers identified in the opo locus. Full size table Analysis of regulatory inputs on the H6_10137 enhancer Taking into account the key role of opo during eye development, we focused our attention on the eye-specific enhancer H6_10137. To analyse its potential regulatory inputs, we scanned for conserved TF-binding sites using the alignment tool MultiTF at ECR browser [46] . 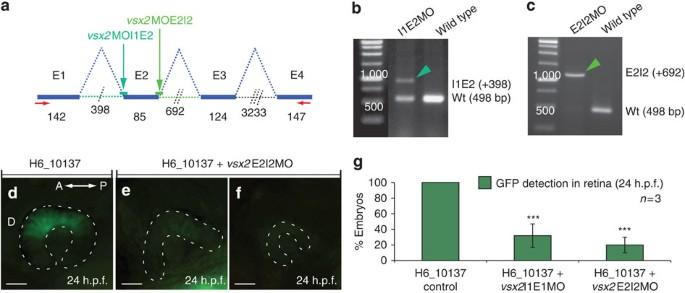Figure 4:Vsx2knockdown using splicing morpholinos. (a) Representation of the zebrafishvsx2transcript from Exon 1 to Exon 4 (E1–E4), introns are depicted as dashed lines; the length of both introns and exons is represented above. RT–qPCR primers are shown as red arrows. The relative positions of theVsx2_MOsare indicated by green bars and arrows. (b,c) Agarose gels showing the aberrant splicing products induced by the morpholinos, as detected by RT–qPCRs. cDNAs from bothvsx2MOs injected embryos and control wild-type embryos were examined at 24 h.p.f. The gels show the morphants’ aberrant transcripts with the inclusion of Intron 2 in E2I2MO (+692 bp) and Intron 1 in I1E2MO (+398 bp). In both conditions, the amount of native transcript (Wt: 498 bp) is reduced when compared with the controls; however, the reduction is more evident in the E2I2 morphant embryos. (d–f) Injection ofVsx2MOsin the lineTg(H6_10137:eGFP). Note that the GFP activity of H6_10137 is reduced in thevsx2morphant embryos when compared with the controls (retina is marked with a dashed line). Scale bar, 50 μm. (g) GFP detection in morphant embryos is significantly reduced when compared with the controls, as determined by the Student’st-test analysis (Pvalue <0.0001). Three independent injection experiments were carried out for a total number of scored embryos of: controls (n=120), H6_10137+ vsx2I1E2MO (n=179) and H6_10137+vsx2E2I2MO (n=25). Error bars indicate s.d. of the mean. The resulting list of putative regulators ( Supplementary Table 4 ) was further filtered to examine their reported developmental expression patterns in The Zebrafish Model Organism Database [47] . This approach revealed a number of TFs expressed in the retinal tissue, such as vsx2 , crx , brca or pbx . Among them, the homeobox TF vsx2 shows an early and specific expression in the neural retina but not in the RPE [12] , [16] , thus resembling most the spatiotemporal activation of H6_10137 ( Fig. 3a,a′ ). Manual ClustalX alignment of the enhancer region for several vertebrate species confirmed the conservation of the consensus binding site for vsx2 (ref. 14 ) detected by multiTF (BS1:142–151 bp), and identified a second conserved site (BS2: 678–687 bp) not initially detected using the default parameters of the algorithm ( Fig. 3b,c ). Figure 3: Identification of Vsx2-binding sites in H6_10137. ( a , a′ ) Confocal section shows GFP expression driven by the H6_10137 enhancer in the neural retina. (l) lens, (nr) neural retina and (rpe) RPE. ( b ) Positional weight matrix showing Vsx2-binding motif. Both Vsx2 DNA-binding sites (BS1 and BS2) located within the H6_10137 sequence are represented. ( c ) Multispecies alignment of H6_10137 enhancer showing sequence conservation of BS1 and BS2 (Human—NCBI36/hg18; Mouse—NCBI37/mm9; Xenopus—JGl 4.2/xenTro3; Medaka—MEDAKA1/oryLat2). ( d ) Both Vsx2 DNA-binding sites were mutated generating the construct mutH6_10137 ( e ) H6_10137 mosaic transgenic embryo (F0) expressing GFP in retina neuroblasts (arrowheads). ( f ) mutH6_10137 transgenic embryo (F0) showing no GFP activity in the retina. ( e′,f′ ) RFP trangenesis controls were observed for both constructs in the heart and somites at 48 h.p.f. (arrowheads). ( g ) Percentages of GFP retina cells for both H6_10137 and mutH6_10137 constructs and its respective controls. Four independent experiments were carried out for a total number of scored embryos injected with the control (H6_10137, n =580) or the mutated (mutH6_10137, n =580) constructs. Error bars indicate s.d. of the mean. Scale bar, 50 μm in ( a , a′ , e , f ) and 100 μm in ( e′,f′ ). Full size image The presence of these conserved binding sites suggests a possible interaction between the TF Vsx2 and the opo H6_10137 enhancer, which is also consistent with both being expressed specifically at the neural retina domain. To investigate whether the identified Vsx2 BS1 and BS2-binding sites are required for the activity of the H6_10137 enhancer, both binding sites were mutated ( Fig. 3d ). The regulatory potential of the mutated enhancer mutH6_10137 (that is, its capacity to drive GFP expression into retina progenitors) was then compared with that of H6_10137 in transient transgenic assays (F0) in zebrafish. As positive transgenesis control, RFP expression controlled by the cardiac-actin:RFP cassette was examined in the somites and heart, and thus the presence of GFP-positive clones in the retina was scored only in RFP-positive embryos ( ∼ 20% of the injected embryos). While 42% of potential founders (that is, RFP-positive embryos) injected with the H6_10137 construct showed typically elongated neuroblasts expressing GFP in the retina at 24 h.p.f., embryos injected with the mutated construct mutH6_10137 did not show any GFP-positive cells in this tissue ( Fig. 3e–g ). Therefore, the mutation of Vsx2 consensus binding sites in the opo eye enhancer abolishes its activity in neural retina precursors, suggesting that Vsx2 may act through this sequence as a direct regulator. Vsx2 regulates opo through binding to the H6_10137 enhancer We reasoned that if the activity of the H6_10137 element in the retina depends on Vsx2 binding, then the loss of vsx2 function should affect the enhancer’s function and hence the expression levels of opo . To address this point, we designed morpholino oligonucleotides aimed to knockdown vsx2 expression in zebrafish. Two splicing morpholino oligonucleotides were designed—I1E2MO and E2I2MO—affecting the splicing of introns 1 and 2, respectively ( Fig. 4a ), and injected into zebrafish embryos at the one-cell stage. Both morpholinos efficiently interfered with splicing at the targeted intron-exon boundaries and significantly reduced the levels of wild-type transcripts, as assessed by quantitative reverse transcription-PCR (RT–qPCR) amplification from morphant embryos’ complementary DNA (cDNA; Fig. 4b,c ). Sequencing of the aberrant transcripts confirmed the intron retention events (that is, of intron 1 and 2, respectively, for I1E2MO and E2I2MO) and consequently, the splicing disruption of vsx2 mRNA in the morphants. Figure 4: Vsx2 knockdown using splicing morpholinos. ( a ) Representation of the zebrafish vsx2 transcript from Exon 1 to Exon 4 (E1–E4), introns are depicted as dashed lines; the length of both introns and exons is represented above. RT–qPCR primers are shown as red arrows. The relative positions of the Vsx2_MOs are indicated by green bars and arrows. ( b , c ) Agarose gels showing the aberrant splicing products induced by the morpholinos, as detected by RT–qPCRs. cDNAs from both vsx2 MOs injected embryos and control wild-type embryos were examined at 24 h.p.f. The gels show the morphants’ aberrant transcripts with the inclusion of Intron 2 in E2I2MO (+692 bp) and Intron 1 in I1E2MO (+398 bp). In both conditions, the amount of native transcript (Wt: 498 bp) is reduced when compared with the controls; however, the reduction is more evident in the E2I2 morphant embryos. ( d – f ) Injection of Vsx2MOs in the line Tg(H6_10137:eGFP) . Note that the GFP activity of H6_10137 is reduced in the vsx2 morphant embryos when compared with the controls (retina is marked with a dashed line). Scale bar, 50 μm. ( g ) GFP detection in morphant embryos is significantly reduced when compared with the controls, as determined by the Student’s t -test analysis ( P value <0.0001). Three independent injection experiments were carried out for a total number of scored embryos of: controls ( n =120), H6_10137+ vsx2I1E2MO ( n =179) and H6_10137+vsx2E2I2MO ( n =25). Error bars indicate s.d. of the mean. Full size image We then evaluated the effect of vsx2 knockdown on H6_10137 activity by injecting these morpholinos into one-cell-stage transgenic embryos from the stable line Tg(H6_10137:eGFP) . Injection of both morpholinos resulted in conspicuous morphological eye defects, which will be discussed in the next section, and caused a dramatic decrease of the levels of GFP signal in the transgenic embryos at 24 h.p.f. ( Fig. 4d–f ). GFP signal could only be detected in 20–30% of the injected embryos ( Fig. 4g ). These results indicate that a reduction of functional vsx2 in the neural retina negatively impinges on the regulatory capability of H6_10137, suggesting that vsx2 acts as a positive regulator of the opo gene. To test this possibility, we examined both in vsx2 gain- and loss-of-function conditions the expression of opo by RT–qPCR. The injection of I1E2MO and E2I2MO morpholinos in zebrafish embryos, both separately or in combination, strongly reduced opo levels in a dose-dependent manner, as determined by RT–qPCRs ( Fig. 5a,b ) in 24-h.p.f. samples. This reduction became even more evident when only the heads of knockdown embryos were used as source material for the RT–qPCRs ( Fig. 5b ). Conversely, the injection of zebrafish vsx2 RNA (100 and 300 ng μl −1 ) into one-cell embryos resulted in a dose-dependent enhancement of opo expression ( Fig. 5c ). Taken together, these results show that vsx2 is a positive regulator of opo . ChIP followed by quantitative PCRs (ChIP–qPCR) assays confirmed that this regulation is exerted through direct binding of Vsx2 to the H6_10137 enhancer. Indeed, RNA injection of a functional tagged GFP_Zvsx2 fusion ( Fig. 5d ) followed by pull down using anti-GFP antibodies, enabled determining a significant enrichment in the ChIP sample of the endogenous zebrafish enhancer (that is, the homologous region to the human H6_10137 fragment) when compared with the housekeeping gene ef1a , used as a negative control ( Fig. 5e ). This enrichment in the ChIP sample was even higher than the observed for a fragment of the vsx1 _promoter, previously identified as a Vsx2 direct target [48] ( Fig. 5e ). Therefore, these results indicate that the H6_10137 enhancer is a direct target of the TF Vsx2. 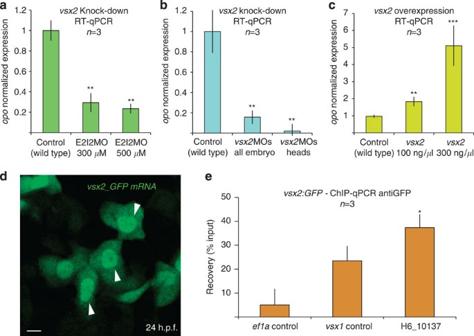Figure 5:Vsx2regulatesopoexpression and binds directly to H6_10137 enhancer. (a,b) Quantification ofopoexpression levels by RT–qPCR show thatopoexpression is significantly reduced invsx2morphant embryos (24 h.p.f.) in a dose-dependent manner (n=3). (b) The reduction ofopoexpression is more pronounced when only the heads of co-injected embryos with bothvsx2MOs were used for the quantification (n=3). (c) The quantification of expression levels in embryos injected withvsx2RNA shows thatopoexpression is significantly higher than in controls (n=3). (d) Confocal microscopy image of epidermal cells of an embryo injected with vsx2GFP RNA. Thevsx2GFPRNA fusion protein localizes at the nuclei (arrowheads) at 24 h.p.f. Scale bar, 5 μm. (e) ChIP experiments were performed using chromatin extracts from dissected heads fromvsx2GFPRNA injected embryo and an anti-GFP antibody. In qPCRs, the recovery of the H6_10137 sequence was significantly increased when compared to the negative control (ef1a). Error bars indicate s.e.m. from three independent ChIP/qPCR experiments. One-way analysis of variance was used to evaluate the statistical significance. Figure 5: Vsx2 regulates opo expression and binds directly to H6_10137 enhancer. ( a , b ) Quantification of opo expression levels by RT–qPCR show that opo expression is significantly reduced in vsx2 morphant embryos (24 h.p.f.) in a dose-dependent manner ( n =3). ( b ) The reduction of opo expression is more pronounced when only the heads of co-injected embryos with both vsx2 MOs were used for the quantification ( n =3). ( c ) The quantification of expression levels in embryos injected with vsx2 RNA shows that opo expression is significantly higher than in controls ( n =3). ( d ) Confocal microscopy image of epidermal cells of an embryo injected with vsx2GFP RNA. The vsx2GFP RNA fusion protein localizes at the nuclei (arrowheads) at 24 h.p.f. Scale bar, 5 μm. ( e ) ChIP experiments were performed using chromatin extracts from dissected heads from vsx2GFP RNA injected embryo and an anti-GFP antibody. In qPCRs, the recovery of the H6_10137 sequence was significantly increased when compared to the negative control ( ef1a ). Error bars indicate s.e.m. from three independent ChIP/qPCR experiments. One-way analysis of variance was used to evaluate the statistical significance. Full size image Vsx2 knockdown impairs optic cup folding To further corroborate the role of vsx2 in eye morphogenesis, the morpholinos I1E2MO and I2E2MO were injected in a transgenic Tg(vsx2.2 :GFPcaax) background. In this line, the membranes of the neural retina precursors are specifically labelled facilitating morphological observations. The analysis of the resulting morphants revealed a similar range of ocular malformations for each morpholino ( Supplementary Table 5 ). A reduction of the eye size (microphthalmia) and optic cup folding defects were observed in 66 and 57% of the I1E2MO and E2I2MO morphants, respectively ( Fig. 6a–c, a′–c′ ). In addition, most severely affected embryos (12 and 15% of the I1E2MO and E2I2MO morphants, respectively) displayed anophthalmia ( Fig. 6d,d′ ). These defects were specific since the co-injection of vsx2 RNA and morpholino E2I2MO increased the percentage of embryos phenotypically classified as wild type (73 versus 28% in E2I2MO-injected embryos; Fig. 6e ). In agreement with our observations ( Fig. 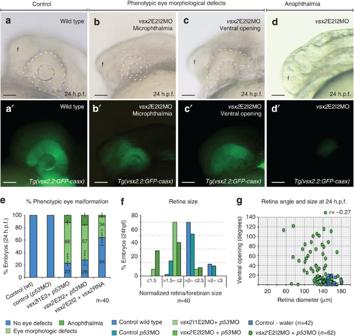Figure 6: Eye morphological defects ofvsx2morphant embryos. (a-a’) Wild-type control embryos showing no eye defects; (b-c’) Morphological eye defects ofvsx2morphants embryos (retinas are marked with a dashed line).Vsx2morphant embryos displaying microphthalmia (b-b’) and ventral opening of the retina (c-c’). (d-d’)vsx2morphant embryos showing anophthalmia (e) % of phenotypic eye malformations in control andvsx2morphant embryos. Note that in co-injected embryos with E2I2MO andvsx2mRNA, the ocular malformations were significantly reduced when compared with embryos injected only with E2I2MO. Error bars indicate standard deviation. One-way analysis of variance was used to evaluate the statistical significance (f) Distribution of relative retinal size in control andvsx2morphants (g) Correlation between ventral opening angle and diameter in retinae from both controls andvsx2morphant embryos. Note the low Pearson correlation coefficient (r=−0.27) between these two parameters. Scale bar=50 μm. 6F and Supplementary Table 6 ), microphthalmia has already been described in vsx2 loss-of-function models in both mouse and zebrafish [13] , [16] . Moreover, at optic cup stages, morphant retinas showed reduced cell number without exhibiting increased cell death (that is, pyknotic nuclei) or significant variation of the mitotic index ( Supplementary Fig. 2 ). These observations suggest an extended M/G1 phase in the morphant retinas, as previously demonstrated in Vsx2 -mutant mice [49] . Figure 6: Eye morphological defects of vsx2 morphant embryos. ( a - a’ ) Wild-type control embryos showing no eye defects; ( b - c’ ) Morphological eye defects of vsx2 morphants embryos (retinas are marked with a dashed line). Vsx2 morphant embryos displaying microphthalmia ( b - b’ ) and ventral opening of the retina ( c - c’ ). ( d - d’ ) vsx2 morphant embryos showing anophthalmia ( e ) % of phenotypic eye malformations in control and vsx2 morphant embryos. Note that in co-injected embryos with E2I2MO and vsx2 mRNA, the ocular malformations were significantly reduced when compared with embryos injected only with E2I2MO. Error bars indicate standard deviation. One-way analysis of variance was used to evaluate the statistical significance ( f ) Distribution of relative retinal size in control and vsx2 morphants ( g ) Correlation between ventral opening angle and diameter in retinae from both controls and vsx2 morphant embryos. Note the low Pearson correlation coefficient ( r =−0.27) between these two parameters. Scale bar=50 μm. Full size image Besides size reduction, we also observed that morphant retinas remained ventrally opened at 24 h.p.f., when the folding of the optic cup is already completed in control embryos ( Fig. 7a–f ). To analyse this phenomenon quantitatively, aperture angles were measured at 24 h.p.f. in more than 100 embryos per morpholino. This analysis revealed that around 70% of vsx2 -knockdown embryos displayed ventral clefts ranging from 21° to 120°, whereas the range ventral opening in control embryos was between 0° and 20° ( Fig. 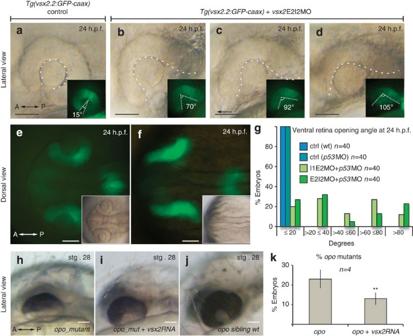Figure 7:Vsx2morphants: ventral aperture retina phenotype quantifications. Control wild-type embryos in (a,e) andvsx2morphant embryos in (b–d,f) showing ocular morphology. Dashed lines indicate the angle of the ventral opening of the retinae for each embryo.Vsx2morphant embryos show large ventral apertures at 24 h.p.f., when compared with the control embryos. (g) Quantification of the ventral apertures in thevsx2morphant embryos (9 ng ofvsx2MO mixed with 4 ng ofp53MO, per embryo) and its respective controls at 24 h.p.f. (h) Eye morphology ofopomutant in medaka at stage 28. (i) Eye morphology of opomutant injected with 200 pg per embryo ofvsx2RNA shows a reduction of the ventral opening. (j) Eye morphology of wild-type sibling showing no eye phenotype. (k) Quantification of the % of embryos displaying an ocular phenotype in the progeny ofopocarriers both uninjected (opo,n=280), and injected withvsx2RNA (opo+vsx2RNA)n=61). Student’st-test analysis (Pvalue <0.005). Scale bar, 50 μm. 7g ; Supplementary Table 7 ). Interestingly, although reduced retinal size and folding defects coexist frequently in the morphant retinas, no significant correlation between these two parameters was observed ( Fig. 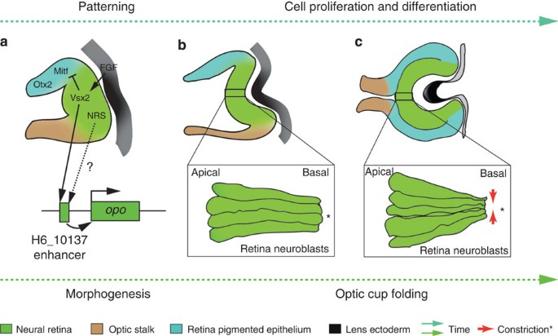Figure 8: Proposed model for vsx2-coordinated coupling between neural retina patterning and morphogenesis (a) During optic vesicle stages,vsx2is required to establish neural retina identity, by suppressing RPE specifiers such asmitf. Our work shows that at this stage, vsx2 binds to the H6_10137 enhancer and regulatesopotranscription levels. Potential regulatory activity of other neural retina specifiers (NRS) on the H6_10137 element has also been depicted. (b,c) During optic cup folding,opois required for basal constriction of the neuroblasts’ feet *28, whilevsx2maintains the proliferative state and identity of the retinal domain. 6g and Supplementary Table 8 ). Taken together, these results point to an essential role for vsx2 during the folding of the optic cup in zebrafish. Figure 7: Vsx2 morphants: ventral aperture retina phenotype quantifications. Control wild-type embryos in ( a , e ) and vsx2 morphant embryos in ( b – d,f ) showing ocular morphology. Dashed lines indicate the angle of the ventral opening of the retinae for each embryo. Vsx2 morphant embryos show large ventral apertures at 24 h.p.f., when compared with the control embryos. ( g ) Quantification of the ventral apertures in the vsx2 morphant embryos (9 ng of vsx2 MO mixed with 4 ng of p53 MO, per embryo) and its respective controls at 24 h.p.f. ( h ) Eye morphology of opo mutant in medaka at stage 28. ( i ) Eye morphology of o po mutant injected with 200 pg per embryo of vsx2 RNA shows a reduction of the ventral opening. ( j ) Eye morphology of wild-type sibling showing no eye phenotype. ( k ) Quantification of the % of embryos displaying an ocular phenotype in the progeny of opo carriers both uninjected ( opo , n =280), and injected with vsx2 RNA ( opo + vsx2 RNA) n =61). Student’s t -test analysis ( P value <0.005). Scale bar, 50 μm. Full size image To further investigate the epistatic relationship between vsx2 and opo , we took advantage of the hypomorphic condition of the opo mutation in medaka (that is, 20% of the wild-type protein is still synthetized) [28] . We tested whether vsx2 overexpression could rescue opo ocular phenotype by injecting zebrafish vsx2 RNA into one-cell-stage medaka embryos derived from opo heterozygous crosses. Similar to our results in zebrafish, the injection of vsx2 RNA in medaka embryos (200 ng μl −1 ) also resulted in an enhancement of opo expression ( Supplementary Fig. 3 ). Moreover, the predicted rescue was observed as a significant reduction in the percentage of injected embryos showing an ocular malformation phenotype ( Fig. 7h–j ). On injection of vsx2 RNA, the percentage of embryos displaying the characteristic large ventral opening was reduced from an approximately Mendelian proportion, 23.9±3.7%, as expected from a carriers’ cross, to 15,4±4.8% ( Fig. 7k and Supplementary Table 9 ). This result confirms the role of vsx2 as an upstream regulator of opo function during optic cup folding. In this work, we have provided a comprehensive study of the regulatory landscape harbouring the morphogenetic gene opo . Within the large syntenic block that comprises slc35b3 , opo and tfap2a ( ∼ 2 Mb in humans), we have analysed a smaller domain (1.5 Mb in human genomes) that includes both opo and tfap2a. This genomic area is flanked by CTCF-binding sites [50] and contains the enhancers identified in our analysis. The fact that opo and tfap2a are not separated by CTCF-binding sites and that they are both contained within the same topologically associating domain [51] open the possibility that common cis -regulatory elements may co-regulate these two genes. Indeed, opo and tfap2a may constitute a small synexpression cluster in the genome, given their common expression in neural crest derivatives and their role in craniofacial development [28] , [52] . Here we have used a combination of phylogenetic footprinting and predictive epigenetic marks to identify candidate cis -regulatory regions (that is, CNEs and active enhancers, respectively), which were then functionally tested in transgenesis assays in zebrafish. Although this is a systematic approach, it is reasonable to consider that the collection of enhancers identified here represents an underestimate of the actual number of regulatory regions in the locus. Some of the CNEs that were unable to activate GFP expression in a reproducible pattern in our assays may either require context-dependent regulatory information or are simply active outside the developmental window considered in this study. In fact, although the tissue domains targeted by the identified enhancers recapitulate most of the opo expression pattern, there are a few opo positive tissues, such as the pronephros and the heart, for which no active enhancers were identified. The definition of cis -regulatory regions within the opo locus is not only relevant to understand the transcriptional regulation of this developmental gene, but may also be important in the context of human hereditary diseases. Sequence variants linked to human diseases are frequently associated to cis -regulatory regions [53] . In fact, among the three translocation break points described within the locus in orofacial cleft patients [37] , the 3′ distal translocation t(6;9)(p24;q22.3) involves a non-coding region that includes several of the conserved enhancers identified in this study. Particularly relevant are the enhancers H6_09516 and H6_09617, which drive the reporter expression in facial derivatives, and hence are candidate regions to be examined further in hereditary orofacial clefting. The H6_10137 region is the only eye-specific enhancer identified in our transgenesis screen of human CNEs in zebrafish. The fact that opo is the only gene expressed early in the retina in the genomic neighbourhood indicates that H6_10137 is an opo enhancer. An equivalent region driving the expression to the developing eye is present in the medaka 5.6-kb proximal element, thus suggesting that the enhancer is not only conserved at sequence level but also functionally in vertebrates. This is in line with what has been observed for a majority of the CNEs comparatively tested in vertebrate species [54] . Here we have identified conserved binding sites for TF Vsx2 in the H6_10137 region, and showed that they are required to direct its regulatory activity to the neural retina domain. Vsx2 has been characterized both as a repressor and a context-specific activator [20] , [55] , [56] . In agreement with its role as a transcriptional activator, our results show that Vsx2 acts as a positive regulator of opo expression in vivo . ChIP–qPCR and morpholino studies demonstrate that Vsx2 can physically bind the H6_10137 enhancer and regulate its activity. Interestingly, the injection of vsx2 RNA into one-cell-stage transgenic embryos from the stable line Tg(H6_10137:eGFP) did not result in the ectopic expression of the reporter beyond the neural retina domain (not shown). This indicates that Vsx2 input is necessary for the activity of the enhancer, but not sufficient to confer tissue specificity to this genomic element. Thus, additional regulatory inputs may act synergistically with Vsx2 to direct the expression of the enhancer H6_10137 to the neural retina. This could happen either through other regulatory regions of the enhancer or via the conserved Vsx2-binding sites. In fact, Vsx2 sites overlap partially with the preferred binding sites of closely related homeodomain proteins from the paired-like class [57] . Therefore, the possibility that other retinal homeodomain proteins different from Vsx2 may regulate the enhancer through these conserved sites cannot be ruled out. This is particularly the case for the homeobox protein Rx, which is also a well-known retinal determinant [58] . Different roles have been proposed for Vsx2 during eye development in vertebrates. This TF was initially identified in mutant mice and human patients as an important regulator of retinal precursors’ proliferation and lineage specification [13] , [14] . Later studies in mice found that Vsx2 played an essential role in the specification of the neural retina domain, mainly by repressing Mitf family members Mitf and Tfec , and hence preventing the activation of the RPE genetic programme [17] , [18] , [20] . A number of knockdown studies in zebrafish have shown that the reported role for Vsx2 in mammals is, at least, partially conserved in teleosts. Thus, small eye phenotypes, abnormal bipolar cell specification and Mitf upregulation have been described in vsx2 -knockdown embryos in zebrafish [15] , [16] , [48] . Interestingly, one of these reports [15] described abnormally shaped eyes displaying a flattened morphology at early stages in zebrafish (24 h.p.f.). This observation is in agreement with our results showing that vsx2 is required during optic cup morphogenesis in zebrafish. The fact that reduced retinal size and folding defects coexist in vsx2 morphant retinas poses the question as to whether the morphological defects we observed on knockdown of vsx2 in zebrafish are due to a proliferation deficiency. In the light of current evidence, this seems an unlikely possibility. Although cell proliferation was initially hypothesized as a cellular mechanism operating during optic cup morphogenesis [59] , more recent reports using DNA synthesis inhibitors have shown that proliferation is largely dispensable for the morphogenesis of the nervous system in Xenopus [60] and of the optic cup in zebrafish [21] . In fact, optic cup invaginates between 16 and 20 h.p.f. in zebrafish, a 4-h period in which only a modest increase in cell number takes place [21] . Moreover, here we show no significant correlation between retinal size and optic cup folding defects on knockdown of vsx2 in zebrafish ( Fig. 6g ), thus suggesting that vsx2 operates through different genetic pathways to control retinal morphology and size. In contrast to our observations, no optic cup morphogenetic defects have been reported in Vsx2-mutant mice ( or J ), despite the range of variability described for this classical mutation [13] , [61] . A couple of alternative explanations may account for this discrepancy. First, Vsx2 may have a variable regulatory weight on the optic cup morphogenetic programme in different vertebrate groups. The fact that Vsx2 sites overlap with the binding sites of closely related homeodomain proteins opens up the possibility that several retinal determination genes cooperate with Vsx2 during optic cup morphogenesis, either through the opo H6_10137 enhancer or by regulating other unidentified morphogenetic genes. These differential regulatory properties may even vary within vertebrates, as optic cup malformations (that is, coloboma) have been reported in families affected with non-syndromic microphthalmia [14] , [62] . In fact, examples of differential input into gene regulatory networks have been already described during optic vesicle patterning in vertebrates. A prominent example is Mitf , which seems to have a smaller regulatory influence in the RPE specification network in zebrafish than in amniotes [63] . Alternatively, as opo / Ofcc1 is a fast-evolving gene, its developmental function may not be conserved in vertebrates. A previous report isolated Opo/Ofcc1 in mouse, described the existence of two different isoforms (A and B, 926 and 786 amino acids, respectively), and characterized the expression of the gene during development [33] . In an attempt to investigate the role of Opo in mouse, a knockout mouse line deleting exons 3 and 4 of the gene was generated [64] . However, this approach left the entire coding sequence of the shorter isoform B intact, and the knockout animals only displayed a very mild phenotype with asymptomatic hyper-γ-glutamyl-transpeptidasemia. A more comprehensive strategy targeting both isoforms will be required to evaluate to which extent the function of this gene is conserved among vertebrates. In conclusion, the systematic analysis presented here of the regulatory input on the opo promoter has identified several conserved tissue-specific enhancers, including the retinal-specific element H6_10137. Our results indicate that vsx2 , acting directly via the H6_10137 enhancer, is an upstream positive regulator of opo . Furthermore, we show an early requirement for vsx2 during optic cup morphogenesis in zebrafish. We propose a model in which Vsx2 acts as a direct transcriptional link between the patterning of the optic vesicle and the morphogenetic effectors mediating the constriction mechanism required for optic cup folding ( Fig. 8 ). This is a relevant link to understand how tissue identity and epithelial morphogenesis are coordinated during the formation of the vertebrate eye. Figure 8: Proposed model for vsx2-coordinated coupling between neural retina patterning and morphogenesis ( a ) During optic vesicle stages, vsx2 is required to establish neural retina identity, by suppressing RPE specifiers such as mitf . Our work shows that at this stage, vsx2 binds to the H6_10137 enhancer and regulates opo transcription levels. Potential regulatory activity of other neural retina specifiers (NRS) on the H6_10137 element has also been depicted. ( b , c ) During optic cup folding, opo is required for basal constriction of the neuroblasts’ feet * [28] , while vsx2 maintains the proliferative state and identity of the retinal domain. Full size image Identification cloning and transgenesis analysis of CNEs A total of 24 conserved CNEs were selected within the opo locus using VISTA Browser [65] and taking as a reference the human genome (NCBI36/hg18) and the default parameters (≥100 bp and ≥70% identity). The presence of predictive epigenetic marks for enhancer activity [66] that overlap opo -associated CNEs was evaluated using available data from human cell lines [41] , [42] and zebrafish embryos [43] . As a reference, four non-conserved elements marked with H3K4me1 and H3K27ac signals in human cell lines were also tested in our enhancer screening. Twenty-three CNEs were amplified from human genome ( Supplementary Table 1 ) and cloned into PCR8/GW/TOPO vector. Individual CNEs were then transferred to the ZED vector [44] using Gateway technology (Invitrogen). The CNE H6_09084 (chr6: 9084162-9086414) could not be cloned, despite multiple attempts. Zebrafish embryos were microinjected at one-cell stage with 3–5 nl of a solution containing 25 nM of each CNE construct and 25 ng μl −1 of Tol2 RNA. A minimum of 300 embryos per CNE was injected. Putative transgenic embryos, as determined by the expression of the internal control of transgenesis ( cardiac-actin:RFP ), were screened for tissue-specific enhancer activity. Fluorescent RNA in situ hybridizations Fluorescence in situ hybridization experiments were preformed as previously described [34] . We used the following primers: 5′-AAGTTGCAGCAGAAGGCTGTGGAG-3′ and 5′-ATTTTGCGGAATTGGTTGAG-3′, a fragment of the opo gene was PCR amplified from zebrafish cDNA (SuperScript VILO cDNA Synthesis Kit; Invitrogen). The PCR products were cloned into pCR 2.1 TOPO TA cloning vector (Invitrogen), linearized with Xba1 and transcribed with SP6 for riboprobe synthesis. The resulting probe was used at a final concentration of 1.5 ng μl −1 . Cloning of the medaka opo promoter region A 5.6-kb region upstream of the medaka opo start site [28] was amplified from medaka genomic DNA by PCR using the primers: 5′-GTCAGCTATCACCGCAGTCGTCA-3′ and 5′-CCTCACTTCCTTGTGCCGACATG-3. The PCR product was cloned into a PCR8/GW/TOPO vector, transferred to the ZED vector and screened for tissue-specific enhancer activity using zebrafish transgenic assays. In silico prediction of TFfactor-binding sites To scan for conserved TF DNA-binding sites within the H6_10137 sequence, we used Mulan alignments and multiTF search tools, available at the ECR browser ( http://ecrbrowser.dcode.org/ ) [67] . The expression pattern of the transcriptional regulators potentially binding the identified motifs was analysed in the ZFIN database ( http://zfin.org/ ) [47] . ClustalX 2.0 (ref. 68 ) was used for multispecies alignments. Site-directed mutagenesis Vsx2 DNA-binding sites were mutated in the H6_10137-ZED construct by PCR, using QuikChange Multisite-Directed Mutagenesis Kit (Agilent technologies). The following mutagenic primers were used for PCR: 5′-CTATTTTACATTTTCTTAATcgcCAAATCTTAATCTTGACTTTAATG-3′ and 5′-CATTATTAGCGGTCTctgCTTGAAGTTATATCAATGTTAGT-3′. Mutagenized vectors were confirmed by sequencing. Both the mutagenic-H6_10137 (mutH6_10137) and the H6_10137 enhancer constructs were then injected in wild-type zebrafish, as described in the first paragraph of the Methods section. The GFP and RFP activity of the injected vectors was assessed in F0 at 24 and 48 h.p.f., respectively. Morpholino injections Two splicing morpholinos directed against zebrafish vsx2 were obtained from Gene Tools: I1E2MO: 5′-TCATCTGAATCTGTAACATGGAGGA-3′ and E2I2MO: 5′-TTTTCTTTAAGCCCACCTGTGTCGT-3′. Both morpholinos were separately injected (8.5–13 ng per embryo) at one-cell stage in wild-type embryos and in the transgenic lines: Tg(H6_10137:eGFP) and Tg(vsx2.2::GFP:caax) . When co-injected, the concentration range used was 6–10 ng for each vsx2 MO. To prevent potential apoptotic effects, a p53 morpholino ( p53 MO: 5′-GCGCCATTGCTTTGCAAGAATTG-3′), was co-injected with vsx2 MOs at a concentration of 4–6 ng per embryo. Control embryos were injected in parallel with water and p53 MO alone. To assess morpholino efficiency, cDNA samples were obtained from control and injected embryos at 24 h.p.f. cDNA samples were then amplified with the following diagnosis primers: I1E2MOfw: 5′-AGCACACTGGACTCCTTCCCCG-3′; E2I2fw 5′-GGGATTAATTGGGCCTGGAGGTAT-3′; I1E2MOrv and E2I2rv: 5′-AGACTCGGGCAGAGGGATAGAGTGA-3′. PCR products were examined by electrophoresis and sequenced to confirm aberrant splicing events induced by the morpholino. Eye phenotype in morphants was examined at 24 h.p.f. using a fluorescent stereoscope (SZX16–DP71, Olympus). GFP levels, ventral opening angles, retina length and forebrain height were quantified using ImageJ1.45q (Wayne Rasband, National Institute of Health, USA). RT–qPCRs qPCR reactions were performed using SsoFast Evagreen Supermix (Bio-Rad) according to the manufacturer’s instructions in a CFX96 real-time C1000 thermal cycler (Bio-Rad). Quantification of opo expression levels in zebrafish was done using a forward primer placed on the second exon: 5′-CGGTCTTCGCTGTAGATGC-3′ and a reverse primer placed on the third exon: 5′-GACGGCGTAGAGGAATAATG-3′. The results were normalized with ef1a , amplified with the following primers 5′-CTTCTCAGGCTGACTGTGC-3′ and 5′-CCGCTAGCATTACCCTCC-3′. In medaka embryos, opo levels were quantified using the following primers: 5′-GGGGGACAATCGTTCATTAGA-3′ and 5′TCAGAAATTCAGCCGACTTGG-3′. β-actin and ef1a , used as internal controls in these experiments, were amplified using primers for β-actin 5′-CAACAGGGAGAAGATGACC-3′ and 5′-CCAGAGTCCATGACGATACCA and ef1a 5′-AAACCCAGAAACACCGAAACA and 5′-CCTCCGCACTTGTAGATCAG. RNA injections Full-length zebrafish vsx2 was amplified from cDNA using the primers 5′-GGACCGACTCGAAAGCAAAG-3′ and 5′-TTAACGCACAAGCCCAAGTC-3′, and cloned into pCS2+ (Addgene). The resulting vector pCS2:zVsx2 was then linearized with NotI and transcribed with mMESSAGE mMACHINE SP6 Kit (Ambion) to synthesize capped RNA. Vsx2 RNA was injected in one-cell-stage embryos (200 pg and 340 pg per embryo), both in medaka and zebrafish. Similarly, the vector pCS2:GFPVsx2 , obtained after in-frame fusion of eGFP to the 5′ sequence of vsx2 in pCS2:zVsx2 , was employed to synthesize capped GFPVsx2 RNA. ChIP detected by qPCR (ChIP–qPCR) The physical interaction between H6_10137 and Vsx2 was tested by ChIP–qPCR using anti-GFP antibodies (Abcam) in zebrafish embryos expressing the fusion protein GFPVsx2 . In brief, wild-type zebrafish embryos were injected at the one-cell stage, (300 pg per embryo) with capped GFPVsx2 RNA. At 24 h.p.f., 300 heads were dissected and fixed in 1% formaldehyde for 15 min at room temperature. After crosslinking, the tissues were washed, sonicated and immunoprecipitated overnight with prebound anti-GFP-Dynabeads (Sigma). Precipitated DNA fragments and control input samples were subjected to DNA extraction with phenol:chloroform:isoamyl alcohol 25:24:1 and washed with 100% ethanol. RT–qPCRs were performed using the following primers: 5′-CAGTGAAGAAGGAAAGCATGG-3′ and 5′-TGCATCTTACAGAAGAAGAGA-3′ for H6_10137; 5′-GTACCGATTTAATACTGTGG-3′ and 5′-CAGTATAGCATACGCTTTTA-3′ for vsx1 (positive control); and 5′-CTCTCAAATCCGGAGATGCT-3′ and 5′-GAAGCTCTCCACACACATGG-3′for Ef1a (negative control). How to cite this article: Gago-Rodrigues, I. et al. Analysis of opo cis -regulatory landscape uncovers Vsx2 requirement in early eye morphogenesis. Nat. Commun. 6:7054 doi: 10.1038/ncomms8054 (2015).